Substrate-mediated band-dispersion of adsorbate molecular states Charge carrier mobilities in molecular condensates are usually small, as the coherent transport, which is highly effective in conventional semiconductors, is impeded by disorder and the small intermolecular coupling. A significant band dispersion can usually only be observed in exceptional cases such as for π-stacking of aromatic molecules in organic single crystals. Here based on angular resolved photoemission, we demonstrate on the example of planar π-conjugated molecules that the hybridization with a metal substrate can substantially increase the delocalization of the molecular states in selective directions along the surface. Supported by ab initio calculations we show how this mechanism couples the individual molecules within the organic layer resulting in an enhancement of the in-plane charge carrier mobility. Efficient charge transport in organic semiconductors is crucial for their performance despite the fact that the fundamental mechanisms and their dependence on structural properties lack in general a comprehensive understanding. In most scenarios, thermally activated hopping dominates in disordered organic layers, whereas band transport only occurs in well-ordered crystals at low temperatures resulting in much larger charge carrier mobilities [1] , [2] , [3] , [4] , [5] , [6] . Several experimental and theoretical publications address the formation of Bloch-like states in organic materials, but a significant band dispersion is only observed for aromatic condensates with extended π-systems. There, the band width can be of the order of some 100 meV along the π-stacks [7] , [8] , [9] , [10] , [11] , [12] , [13] , [14] , [15] , while it is much smaller in other directions [9] , [16] . It is moreover well-established that the bonding to a metal substrate can lead to new states at the interface because of hybridization between metal and molecular wave functions [17] , [18] . It is an intriguing aspect of this hybridization of localized molecular with delocalized substrate states that it may lead to a lateral delocalization of the resulting hybrid states. Several studies address this issue, but so far the investigated states are exclusively from or at least strongly dominated by features originating from the metal substrate [19] , [20] , [21] , [22] , [23] , [24] , [25] . The strongly dispersing Shockley state can be observed shifted in energy and backfolded because of the adlayer superstructure [19] , [20] , [21] , [25] . A mixing with molecular states could so far not be quantified [22] , [23] . In this article, we show that for ordered layers of flat-lying, planar molecules a substantial delocalization of molecular derived states in the lateral direction occurs owing to the bonding to the substrate. For the model systems 3,4,9,10-perylene-tetracarboxylic-dianhydride (PTCDA) and 1,4,5,8-naphthalene-tetracarboxylic-dianhydride (NTCDA) adsorbed on Ag(110) surfaces the lowest unoccupied molecular orbital (LUMO), which hybridizes with substrate states and is occupied by charge transfer from the metal [26] , [27] , [28] , shows a dispersion of 230 meV and 180 meV, respectively, along the surface in angle-resolved photoelectron spectroscopy (ARPES). Density functional theory (DFT) calculations quantitatively confirm the experimentally observed dispersion and reveal its origin as being primarily due to molecule-metal hybridization. Moreover, temperature-dependent experiments exhibit changes in the LUMO band width, which can be associated with changes in the interfacial bonding strength, thus supporting our finding of a substrate-mediated intermolecular coupling, which leads to a two-dimensionally delocalized wave function of the LUMO-derived interface state. 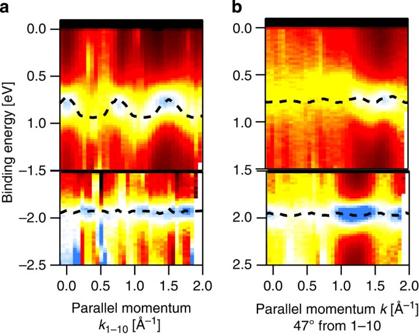Figure 1: Angle-resolved photoemission data of the PTCDA brickwall layer on Ag(110) recorded atT=45 K. (a) Along the ()-direction of the substrate and (b) 47° rotated against the -direction. The dashed black curves represent the dispersion of the LUMO and of the HOMO as calculated by density functional theory (seeFig. 2b. The horizontal line at binding energy EB=1.5 eV indicates a change in the normalization procedure between the LUMO and the HOMO region (seeSupplementary Note 1for details). Experimental evidence for a dispersive band at the interface Figure 1 shows ARPES measurements of the frontier orbitals recorded for one monolayer of PTCDA adsorbed on Ag(110) in the brickwall phase at a sample temperature of 45 K (see Fig. 3 for molecular structure and arrangement in the brickwall layer) [29] , [30] . For panel (a), the measurements were performed along the substrate ( ) direction, that is, from the centre of the Brillouin zone to the intensity maximum of the LUMO [27] , [28] , [31] (see Supplementary Fig. S1 and Supplementary Note 1 ), while the data in Fig. 1b were recorded in a direction rotated by 47° against the ( ) direction. Owing to the strong orbital-specific intensity variations [27] , [28] , [31] the data were normalized as specified in Supplementary Note 2 and Supplementary Fig. S2 . Along ( ) one can clearly identify a periodic variation in the binding energy of about 230 meV for the PTCDA LUMO, which is centred at about 0.8 eV. The energy dispersion thus displays the Bloch-character of the PTCDA LUMO, while the angle-dependent intensity distribution ( Supplementary Fig. S1 ) shows its molecular origin [27] , [28] , [31] . Figure 1: Angle-resolved photoemission data of the PTCDA brickwall layer on Ag(110) recorded at T =45 K. ( a ) Along the ( )-direction of the substrate and ( b ) 47° rotated against the -direction. The dashed black curves represent the dispersion of the LUMO and of the HOMO as calculated by density functional theory (see Fig. 2b . The horizontal line at binding energy E B =1.5 eV indicates a change in the normalization procedure between the LUMO and the HOMO region (see Supplementary Note 1 for details). Full size image The highest occupied molecular orbital (HOMO), which can be observed at a binding energy of about 2.0 eV [27] , [28] , [31] , shows a much smaller energy dispersion of <50 meV. Such small values are well-known from other ARPES measurements on various systems [10] , [15] . Comparing the dispersion along different directions in Fig. 1a , we see that the LUMO disperses highly anisotropically and that its band width is below 70 meV in case of Fig. 1b . Theoretical modelling of the dispersing PTCDA LUMO To further investigate the nature of the observed dispersion, we performed DFT calculations. In a first step we calculated the band dispersion of the PTCDA LUMO and HOMO for a free standing layer of flat-lying molecules using a molecular arrangement identical with the experimentally found lateral positions in the brickwall phase on Ag(110) with slightly bent molecules [32] . 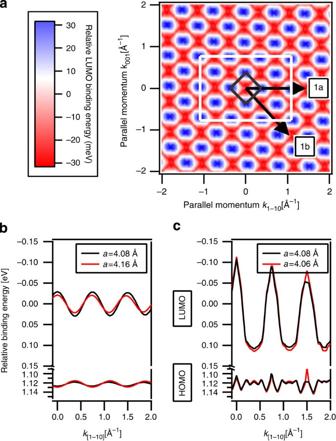Figure 2: Density functional theory calculation of the LUMO and HOMO dispersion in a brickwall PTCDA layer. (a) Theoretical LUMO binding energy distribution over momentum space, calculated for a free standing PTCDA layer. The grey rectangle indicates the PTCDA Brillouin zone, the white rectangle the substrate surface Brillouin zone. The black arrows indicate the directions of the measurements shown inFig. 1a). (b) Binding energy of the LUMO and HOMO of a free standing PTCDA layer as a function of parallel momentum in the ()-direction. (c) Analogous calculation for a PTCDA layer adsorbed on a four layer thick Ag(110) slab. The calculation was performed for different Ag lattice constanta(see legend), thus mimicking a temperature-dependent lattice expansion of the substrate. Figure 2a shows the LUMO dispersion in the k x − k y -plane in an extended Brillouin zone scheme. This illustrates that the dispersion is laterally strongly anisotropic. The black arrows indicate the substrate’s ( )-direction and 47° rotation against the ( ) direction, where strong and weak dispersion occurs, respectively. Although this straightforwardly explains the strong difference in the observed band widths seen in Fig. 1 , the size of the band dispersion is severely underestimated by these free-standing layer calculations. As presented in Fig. 2b , the LUMO (HOMO) band width along () is only about 60 meV (15 meV), which is four times smaller than the experiment shows. This changes dramatically, if, in a second step, we take into account the substrate by placing the monolayer on top of a Ag(110) slab consisting of four atomic layers. The resulting band dispersions along ( ) are shown in Fig. 2c . Although the HOMO band width is only slightly affected by the substrate, the LUMO dispersion is enhanced by a factor of four. This is also reflected in a reduction of the effective hole mass from m eff =3.9 m e for the free-standing layer to m eff =1.1 m e for the monolayer adsorbed on Ag(110) when evaluated at the Γ-point in a parabolic approximation or within a tight-binding fit. Thus, our calculations reveal an increase of the lateral charge carrier mobility in the LUMO state by approximately four times due to the molecule–substrate interaction. Figure 2: Density functional theory calculation of the LUMO and HOMO dispersion in a brickwall PTCDA layer. ( a ) Theoretical LUMO binding energy distribution over momentum space, calculated for a free standing PTCDA layer. The grey rectangle indicates the PTCDA Brillouin zone, the white rectangle the substrate surface Brillouin zone. The black arrows indicate the directions of the measurements shown in Fig. 1a ). ( b ) Binding energy of the LUMO and HOMO of a free standing PTCDA layer as a function of parallel momentum in the ( )-direction. ( c ) Analogous calculation for a PTCDA layer adsorbed on a four layer thick Ag(110) slab. The calculation was performed for different Ag lattice constant a (see legend), thus mimicking a temperature-dependent lattice expansion of the substrate. Full size image Origin of the delocalized state These findings are not entirely unexpected as it is a well-known fact that the bonding of PTCDA to Ag-substrates leads to a hybridization of the LUMO with Ag-sp-states [26] , [27] . The mixing of the localized molecular wave function with the delocalized metal states then also implies a stronger intermolecular coupling within the PTCDA adlayer, and consequently the band dispersion of the LUMO is substantially enhanced. The behaviour of the HOMO is also consistent with this interpretation as it does not show a significant hybridization on Ag-substrates [26] , [27] and thus its lateral band dispersion remains unaffected upon adsorption. To further illustrate this picture, we show partial charge densities calculated around the HOMO and LUMO energies in Fig. 3 (for an additional 3D plot see Supplementary Fig. S3 ). On the one hand, the data are represented as iso-surface plots (purple colour), which highlights the molecular character of the HOMO and LUMO states, respectively. 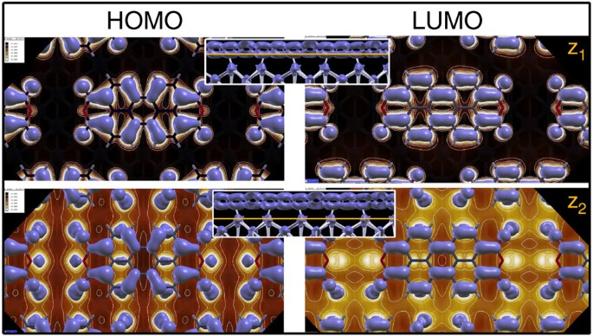Figure 3: Real space model of the PTCDA/Ag(110) brickwall layer. The iso-surfaces in purple show the partial charge density of the HOMO (left) and LUMO (right). Additionally horizontal cuts through the partial charge density visualize the delocalization of the LUMO within distinct planes specified in the two inset graphs (black indicates no, white high partial charge density). In the molecular plane (top panel) no delocalization occurs, contrary to the topmost Ag-plane (bottom panel) showing a significant delocalization. Figure 3 also shows two cuts through the partial charge density in planes parallel to the surface, one close to the molecular plane (top row) and the other near to the topmost Ag-layer (bottom row). Although in the former plane, no significant intermolecular charge overlap of the HOMO and LUMO densities is visible, a significant charge delocalization can be observed close to the surface, which is clearly more pronounced for the LUMO thus emphasizing the role of the substrate in the observed band dispersions. Figure 3: Real space model of the PTCDA/Ag(110) brickwall layer. The iso-surfaces in purple show the partial charge density of the HOMO (left) and LUMO (right). Additionally horizontal cuts through the partial charge density visualize the delocalization of the LUMO within distinct planes specified in the two inset graphs (black indicates no, white high partial charge density). In the molecular plane (top panel) no delocalization occurs, contrary to the topmost Ag-plane (bottom panel) showing a significant delocalization. Full size image Temperature dependence of the band width The strength of the molecule–substrate interaction, and thereby the magnitude of the substrate-enhanced band width of the LUMO, clearly depends on the vertical distance between the molecule and the substrate. In view of several investigations on very similar systems, such as PTCDA/Ag(111) [33] , [34] and NTCDA/Ag(111) [35] , a reduction of this vertical bonding distance can be achieved by lowering the substrate temperature and is accompanied by an energy shift of the LUMO towards larger binding energies. 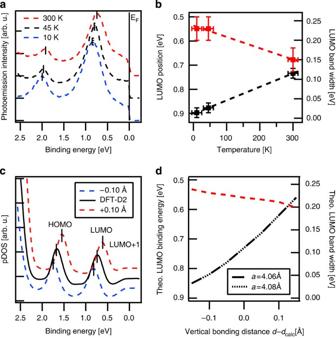Figure 4: Temperature-dependent angle-resolved photoemission data of PTCDA/Ag(110). (a) Energy dispersion curves recorded at temperatures of 300 K (top), 45 K (middle) and 10 K (bottom) atk=1.45 Å−1. The intensity maxima of the LUMO and HOMO are indicated to highlight the shift in energy. (b) LUMO binding energy (black data points) and experimental LUMO band width (red data points) plotted against temperature. (c) Molecule-projected density of states (pDOS) for a PTCDA layer adsorbed on a Ag(110) slab at vertical distances of ±0.10 Å around the density functional theory (DFT) calculation-minimum position. (d) Calculated LUMO binding energy (black curve) for different substrate lattice constantaand band width of the LUMO (red curves) plotted against vertical bonding distance around the DFT-minimum. Figure 4 shows energy distribution curves of PTCDA/Ag(110) recorded in the ( ) direction at k =1.45 Å −1 and thus at the binding energy minimum of the LUMO measured at sample temperatures of 300 K (top), 45 K (middle) and 10 K (bottom). One immediately observes an energy shift of the LUMO and HOMO towards larger binding energies upon decreasing temperature. Note that electron diffraction (see Supplementary Note 3 and Supplementary Fig. S4 ) shows that the lateral order is unchanged by the cooling. When plotting the energy positions of the LUMO maxima against temperature in Fig. 4b , a shift of about 150 meV from T =300 K to T =10 K is revealed. Such a shift is corroborated by the DFT calculations in which the vertical bonding distance has been varied by ±0.1 Å around the DFT-minimum assuming a frozen-in molecular geometry. The resulting molecule-projected density of states curves are shown in Fig. 4c revealing a shift towards larger binding energies upon reducing the vertical distance in agreement with experiment. Figure 4d summarizes these findings and demonstrates that the experimentally observed energy shift of 150 meV is correlated with a change of about 0.1 Å in bonding distance. Note that the influence of substrate screening on the spectral function, in particular on the apparent binding energies of the states, can be estimated from a first-order GW calculation. It is smaller than 100 meV for the distances considered here [36] and is not relevant for the present discussion of the band dispersion. Such a value is very similar to the experimentally observed relation between distance and LUMO position for PTCDA/Ag(111) [33] , [34] . Note that the temperature decrease from 300 to 10 K will also change the substrate lattice constant from 4.084 to 4.069 Å (ref. 37 ), and consequently also the lateral distance between the PTCDA molecules in the adlayer will be reduced. This effect has been considered in our DFT calculations and Fig. 4d shows that this change in lattice constant does not lead to a significant energy shift of the LUMO rendering the change of vertical bonding distance the dominant mechanism. Figure 4: Temperature-dependent angle-resolved photoemission data of PTCDA/Ag(110). ( a ) Energy dispersion curves recorded at temperatures of 300 K (top), 45 K (middle) and 10 K (bottom) at k =1.45 Å −1 . The intensity maxima of the LUMO and HOMO are indicated to highlight the shift in energy. ( b ) LUMO binding energy (black data points) and experimental LUMO band width (red data points) plotted against temperature. ( c ) Molecule-projected density of states (pDOS) for a PTCDA layer adsorbed on a Ag(110) slab at vertical distances of ±0.10 Å around the density functional theory (DFT) calculation-minimum position. ( d ) Calculated LUMO binding energy (black curve) for different substrate lattice constant a and band width of the LUMO (red curves) plotted against vertical bonding distance around the DFT-minimum. Full size image If the lowering of temperature is accompanied by a reduction of the vertical bonding distance, and thereby by an increase of the molecule–substrate hybridization, this should be reflected by an enhanced band width of the LUMO. This is indeed the case as we observe band widths of 150 meV at 300 K and 230 meV at 10 K (red symbols in Fig. 4b ). This finding is reproduced by the DFT calculations, which also yield an increase of the LUMO-projected density of states (red line in Fig. 4d ), thereby resembling the band width of the LUMO dispersion, upon reducing the vertical distance. Although for a quantitative description of the evolution of the LUMO band width a more sophisticated theoretical description including local and nonlocal electron-phonon coupling is needed [6] , this qualitative agreement clearly indicates the influence of the vertical bonding distance on the LUMO band width. Thus, the temperature-dependent ARPES experiment further supports our finding of a substrate-mediated lateral delocalization of the LUMO-derived interface state. Dispersive LUMO band in NTCDA The question remains if this is an effect specific to the PTCDA/Ag(110) system. We can demonstrate the general validity of our finding by the ARPES data of NTCDA on Ag(110) in Fig. 5b , which shows a very similar dispersive character for the LUMO. The planar NTCDA (see molecular structure in Fig. 5a ) also chemisorbs flat lying on Ag(110) resulting in a hybridization and filling of the LUMO. The molecules are arranged in rows [38] in the ( )-direction as illustrated in Fig. 5 , thus the largest band width of 180 meV is observed for the LUMO in this direction. Also in this case, there is a strong enhancement of the LUMO band width from 60 meV for the free-standing layer to 120 meV for the adsorbed monolayer owing to molecule–substrate hybridization. This enhancement of the band width results in a reduction of the effective hole mass from m eff =3.9 m e in the free standing layer to m eff =1.4 m e in the adsorbed layer. Note that the minor deviations in the experimental data around k =0.5 Å −1 are caused by the low ARPES signal of the molecular states and the crossing of the Ag-sp-band. 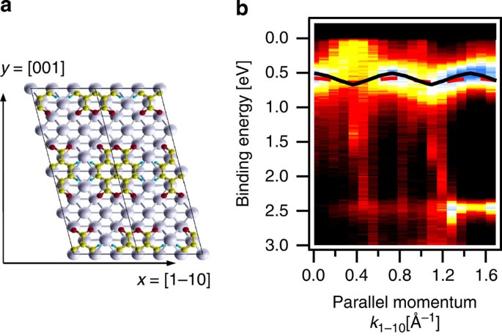Figure 5: The NTCDA brickwall structure. (a) Molecular structure of NTCDA and the arrangement of the molecules on the Ag(110) surface. The photoelectron spectroscopy (PES) data have been measured along the direction marked by the black arrow. (b) Angle-resolved PES data of NTCDA/Ag(110) recorded withhν=36 eV atT=100 K along the ()-direction of the Ag(110) substrate. The dashed red line shows the calculated LUMO dispersion for a free standing layer, the solid black line for a layer adsorbed on a four layer thick Ag slab. Figure 5: The NTCDA brickwall structure. ( a ) Molecular structure of NTCDA and the arrangement of the molecules on the Ag(110) surface. The photoelectron spectroscopy (PES) data have been measured along the direction marked by the black arrow. ( b ) Angle-resolved PES data of NTCDA/Ag(110) recorded with h ν=36 eV at T =100 K along the ()-direction of the Ag(110) substrate. The dashed red line shows the calculated LUMO dispersion for a free standing layer, the solid black line for a layer adsorbed on a four layer thick Ag slab. Full size image On the examples of PTCDA and NTCDA on Ag(110) we have shown that a lateral band dispersion of around 200 meV occurs for the LUMO state in ordered chemisorbed layers of aromatic compounds. The magnitude of this dispersion is of the same order as usually only observed in the π-stacking direction of aromatic molecules. By a comparison with DFT calculations and by temperature-dependent ARPES experiments we have demonstrated that the observed effect can be traced back to a substrate-mediated coupling of the adsorbate molecules. This coupling is based on the hybridization of the LUMO wave function with delocalized Ag-sp-states thus leading to a molecule-metal hybrid state with a significant lateral delocalization. Such a delocalization of the molecular states was investigated by several researchers [19] , [20] , [21] , [22] , [23] , [24] , [25] , [39] , and a substrate-mediated enhancement of lateral band dispersion was interpreted [39] but so far not evidently shown. Moreover, we would like to stress that the intermolecular delocalization reported here is based on the hybridization between molecular and substrate states and is thus clearly different from a mere doping (with, for example, alkali atoms). In the latter case, a similar charge transfer from the dopants to the host molecules occurs, but the coupling between the molecules is not significantly amplified [8] , [40] . A coupling of molecular induced states was also reported [41] , [42] , where the formation of molecular networks leads to quantum wells of the substrate electrons present at the surface that might be backscattered or coupled, but the states of the molecular semiconductor itself are not regarded. Preparation of ultrathin molecular films The experiments were performed in ultrahigh vacuum systems with base pressures of 2 × 10 −10 mbar. The PTCDA and NTCDA films were prepared in attached preparation chambers by organic molecular beam deposition with a deposition rate of 0.2 monolayers per min onto clean and well-ordered Ag(110) single-crystal surfaces [43] at room temperature. Angular resolved photoemission measurements The angle-resolved photoemission measurements for PTCDA/Ag(110) were obtained with monochromatized UV lamps for He I α radiation ( hv =21.22 eV) and high-resolution photoelectron analysers (Scienta SES200 and R4000, respectively). The overall energy resolution was about Δ E =10 meV for both systems. The ARPES data for NTCDA/Ag(110) was recorded at beamline 9 Å of the Hiroshima Synchrotron Radiation Centre using photons with circular polarization and a photon energy hv=36 eV. The beamline is equipped with a 6-axes manipulator (i-GONIO, R-Dec Co.) and a Scienta R4000 photoelectron analyser enabling photoemission measurements with an energy resolution better than 10 meV at a base pressure of 4 × 10 −11 mbar [35] , [38] , [44] , [45] . First-principles calculation Electronic structure calculations are performed within the framework of DFT employing the ab initio total-energy and molecular-dynamics programme VASP (Vienna ab initio simulation programme) developed at the Institut für Materialphysik of the Universität Wien [46] , [47] . The projector augmented waves [48] with a kinetic energy cutoff of 25 Ry, a k -mesh of 8 × 8 × 1, and a first-order Methfessel–Paxton smearing [49] of 0.2 eV has been used. Exchange and correlation effects are treated with the generalized gradient approximation [50] with empirical van-der-Waals corrections [51] . As structural models, we use free-standing layers of PTCDA and NTCDA as well as respective adsorbed monolayers on Ag(110) represented by atomic layers in a repeated slab approach. Before evaluating the electronic structure properties, the geometry has been relaxed starting from experimentally observed adsorption sites and distances. Band dispersions of HOMO and LUMO levels of the free-standing layers are evaluated directly from the Kohn–Sham orbital energies, whereas the respective band dispersions for the adsorbed monolayers are gained from k -resolved molecule-projected density of states curves. Partial charge densities of HOMO and LUMO are obtained by integrating the charge partial densities in a energy window of 0.5 eV centred around the HOMO and LUMO energy positions, respectively. A dditional information How to cite this article: Wießner, M. et al. Substrate-mediated band-dispersion of adsorbate molecular states. Nat. Commun. 4:1514 doi: 10.1038/ncomms2522 (2013).